Light-independent regulation of algal photoprotection by CO2availability 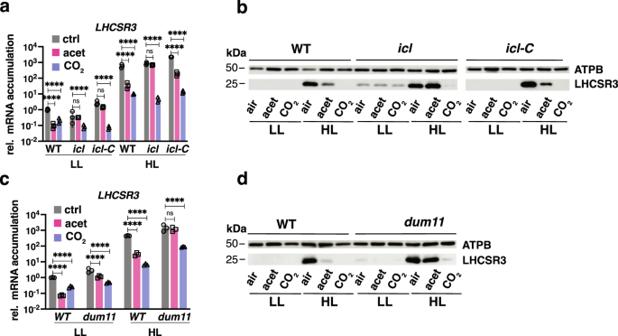Fig. 1: Acetate needs to be metabolized to inhibit LHCSR3 accumulation. WT,icl,icl-Canddum11strains were acclimated for 16 h in LL (15 µmol photons m−2s−1) in HSM; sparged with air (labelled as “air”); sparged with air and supplemented with 10 mM sodium acetate (labelled as “acet”); sparged with air enriched with 5% CO2(labelled as “CO2”). After sampling for the LL conditions, light intensity was increased to 600 µmol photons m−2s−1(HL); samples were taken 1 h (RNA) or 4 h (protein) after exposure to HL.a,c. Accumulation ofLHCSR3mRNA at the indicated conditions normalized to WT LL ctrl (n= 3 biological samples, mean ± s.d.). The p-values for the comparisons of acetate and CO2conditions to air are based on ANOVA Dunnett’s multiple comparisons test of log10 transformed mRNA data as indicated in the graphs (*P< 0.005, **P< 0.01, ***P< 0.001, ****P< 0.0001, ns, not significant). Exact p-values can be found at the Source Data file.b,d. Immunoblot analyses of LHCSR3 and ATPB (loading control) under the indicated conditions. Representative datasets of experiments repeated three times. Photosynthetic algae have evolved mechanisms to cope with suboptimal light and CO 2 conditions. When light energy exceeds CO 2 fixation capacity, Chlamydomonas reinhardtii activates photoprotection, mediated by LHCSR1/3 and PSBS, and the CO 2 Concentrating Mechanism (CCM). How light and CO 2 signals converge to regulate these processes remains unclear. Here, we show that excess light activates photoprotection- and CCM-related genes by altering intracellular CO 2 concentrations and that depletion of CO 2 drives these responses, even in total darkness. High CO 2 levels, derived from respiration or impaired photosynthetic fixation, repress LHCSR3 /CCM genes while stabilizing the LHCSR1 protein. Finally, we show that the CCM regulator CIA5 also regulates photoprotection, controlling LHCSR3 and PSBS transcript accumulation while inhibiting LHCSR1 protein accumulation. This work has allowed us to dissect the effect of CO 2 and light on CCM and photoprotection, demonstrating that light often indirectly affects these processes by impacting intracellular CO 2 levels. A major challenge for photosynthetic organisms is to efficiently acclimate to highly dynamic light and nutrient conditions that occur in natural environments. While light provides the energy that fuels photosynthetic CO 2 fixation, excess light can cause oxidative damage and ultimately result in cell death. Therefore, light absorption must be precisely managed via photoprotective mechanisms that help integrate the use of light energy with CO 2 availability and the potential of the organism to grow and store fixed carbon. A dominant photoprotective mechanism, called qE (energy-dependent quenching), results in the harmless dissipation of excess absorbed light energy as heat [1] , [2] . Triggering qE requires the synthesis of specific proteins and pigments that are controlled both transcriptionally and post-transcriptionally. In the green microalga Chlamydomonas reinhardtii (hereafter Chlamydomonas ), qE depends on the nucleus-encoded, chloroplast-localized Light Harvesting Complex-Stress Related (LHCSR) proteins LHCSR1, LHCSR3 and Photosystem II Subunit S, PSBS, which are present in many algae and lower plants [3] and belong to the Light Harvesting Complex protein superfamily [4] . The LHCSR3.1 and LHCSR3.2 genes in Chlamydomonas encode identical LHCSR3 proteins [5] , while PSBS1 and PSBS2 encode proteins that differ by only one amino acid of the chloroplast transit peptide [6] . While LHCSR1 and LHCSR3 are present in algae but not in vascular plants, PSBS is present in both [4] . PSBS in Chlamydomonas is transiently expressed in cells exposed to high light (HL) [6] , [7] and accumulates in cells exposed to UV-B irradiation [8] . LHCSR3 is the main qE effector protein in HL [5] , although LHCSR1 can significantly contribute to qE under certain conditions [9] . In Chlamydomonas , expression of LHCSR3 has been reported to increase upon absorption of blue-light by the photoreceptor phototropin (PHOT1) [10] and involves calcium ion signaling [11] , active photosynthetic electron transport (PET) [10] , [11] and the transcriptional factor CONSTANS, which is also required for activation of the LHCSR1 and PSBS genes [12] , [13] . Similar to the dynamic light cue, the concentration of inorganic carbon (HCO 3 − , CO 2 and CO 3 2− , together designated Ci) in aquatic environments varies spatially and temporally; aquatic CO 2 levels can also fluctuate from extremely high (hyper-saturated) to extremely low [14] . Because low CO 2 levels limit photoautotrophic growth, microalgae have evolved a CO 2 Concentrating Mechanism (CCM) that elevates the level of CO 2 at the site of fixation by Ribulose-1,5-bisphosphate carboxylase/oxygenase (RuBisCO). Major components of the CCM are carbonic anhydrases (CAH), which facilitate interconversions among the different Ci species, and Ci transporters. The genes encoding many Ci transporters and CAHs are under the control of the zinc-finger type potential transcription regulator CIA5 (also CCM1) [15] , [16] , which is localized in the nucleus [17] and controls expression of low-CO 2 responsive genes. In addition to the use of CO 2 to support phototrophic growth in the light, Chlamydomonas can also use the two-carbon molecule acetate either in the dark to support heterotrophic growth, or in the light, to support photoheterotrophic or mixotrophic growth [18] . Acetate is incorporated into acetyl-CoA either in a one-step reaction catalyzed by acetyl-CoA synthetase (ACS), or in two steps that use acetate kinase (ACK) and phosphate acetyltransferase (PAT), which sequentially catalyze the formation of acetyl-phosphate and acetyl-CoA [19] . 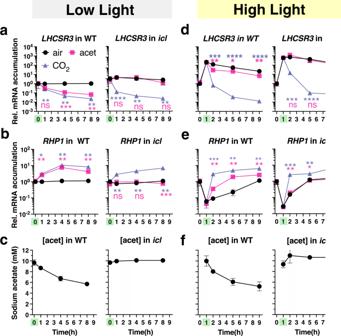Fig. 2: LHCSR3 inhibition is driven by CO2derived from the metabolism of acetate. Experiment at LL:a,bmRNA accumulation ofLHCSR3andRHP1andcconcentration of sodium acetate in the growth medium in WT andiclstrains. Cells were acclimated overnight at LL (15 µmol photons m−2s−1) in HSM sparged with air. At t = 0 cells either continued being sparged with air (labelled “air”); or sparged with air and supplemented with 10 mM sodium acetate (labelled “acet”); or sparged with air enriched with 5% CO2(labelled “CO2”). The addition of acetate or CO2is indicated with a green mark on the x-axis. Samples were taken at t = 0, 1 h, 4 h and 8 h. Experiment at HL:d,emRNA accumulation ofLHCSR3andRHP1andfconcentration of sodium acetate in the growth medium in WT andiclstrains. Cells were acclimated overnight at LL (15 µmol photons m−2s−1) in HSM sparged with air; at t = 0 light intensity was increased to 600 µmol photons m−2s−1. At t = 1 h cells either continued being sparged with air (labelled “air”); or sparged with air and supplemented with 10 mM sodium acetate (labelled “acet”); or bubbled with air enriched with 5% CO2(labelled “CO2”), always at 600 µmol photons m−2s−1. The time of addition of acetate or CO2is highlighted in green on the x-axis. Samples were taken at t = 0, 1 h, 2 h, 5 h and 9 h. (n= 3 biological samples, mean ± s.d.). Thepvalues for the comparisons of acetate and CO2conditions to air (LL; t = 1, 4, 8 h, HL; t = 2, 5, 9 h) are based on ANOVA Dunnett’s multiple comparisons test of log10 transformed mRNA data as indicated in the graphs (*P< 0.005, **P< 0.01, ***P< 0.001, ****P< 0.0001, ns, not significant), following the color-code of the datasets. Exact p-values can be found at the Source Data file. Please note that in some cases the error bars are smaller than the data point symbols. Acetyl-CoA can then enter the glyoxylate cycle, a shunt of the tricarboxylic acid (TCA) cycle [20] , recently characterized in Chlamydomonas [21] , where it can be converted to metabolites that are used for anabolic metabolism. Alternatively, acetyl-CoA enters the TCA cycle to feed the respiratory chain with reducing equivalents. Both, the glyoxylate cycle and respiration are essential for growth in the dark since Chlamydomonas mutants affected in either of these processes are unable to grow heterotrophically [21] , [22] . Despite the evident connection between light and CO 2 levels, the physiological responses to different light and CO 2 availabilities have been traditionally studied separately. However, several lines of evidence indicate that both acetate and Ci abundance impact not only qE but also the establishment of the CCM in Chlamydomonas [23] , [24] , [25] , [26] , while LHCSR3 transcripts accumulation have been reported to be CIA5-dependent [26] , [27] , [28] . Yet, the mechanism(s) associated with carbon-dependent regulation of qE and CCM induction and the intimate link between the two processes have still not been clearly defined. Here, using genetic and mathematical modelling approaches, we demonstrate that inhibition of LHCSR3 accumulation and CCM activity by acetate is at the level of transcription and a consequence of metabolically produced CO 2 . We also show that exposure of Chlamydomonas to HL triggers not only HL responses, but also low-CO 2 responses, and we report the discovery of a novel CO 2 - and CIA5-dependent mechanism that activates LHCSR3 gene expression even in complete darkness. Finally, we propose that PET is critical for the activation of LHCSR3 transcription because it sustains CO 2 fixation, consuming intracellular CO 2 and thereby relieving its inhibitory effect. This work emphasizes the importance of CO 2 in regulating photoprotection and the CCM, and demonstrates that light often indirectly affects these processes by altering intracellular CO 2 levels. CO 2 generated from acetate metabolism inhibits LHCSR3 To gain insights into the effect of carbon metabolism on photoprotection, we explored the impact of acetate and high CO 2 on LHCSR3 mRNA and protein levels in wild-type (WT) cells and in two mutants impaired in acetate metabolism; the icl mutant, which lacks isocitrate lyase, a key enzyme of the glyoxylate cycle [21] , and the dum11 mutant, which is defective in the ubiquinol cytochrome c oxidoreductase (respiratory complex III) [29] . The presence of acetate in the medium of WT cells inhibited the accumulation of the LHCSR3 transcript (Fig. 1a , note the logarithmic scale) in both low light (LL) and high light (HL) conditions. No protein was detected in WT under any condition in LL, but inhibition by acetate was apparent in HL (Fig. 1b ), as previously reported [25] . However, in the icl mutant, acetate had no inhibitory effect on the accumulation of LHCSR3 mRNA (Fig. 1a ) or protein (Fig. 1b ) in either HL or LL, while the icl::ICL -complemented line, designated icl-C , exhibited similar behavior to that of WT cells (Fig. 1a, b ). Additionally, acetate did not alter LHCSR3 transcript or protein accumulation in HL-treated dum11 mutant cells (Fig. 1c, d ), while under LL, acetate inhibited LHCSR3 transcript in the dum11 mutant but to a much smaller extent than in WT (Fig. 1c ) . Together, these results suggest that the acetate administered to the cells must be metabolized for it to have a suppressive effect on the accumulation of LHCSR3 transcript and protein in HL. We also sparged WT, icl, icl-C and dum11 cells with 5% CO 2 both in LL and HL. CO 2 strongly repressed the accumulation of LHCSR3 mRNA and protein in all genotypes, including the metabolic mutants icl and dum11 for which expression of LHCSR3 was unaffected by acetate (Fig. 1a-d ). Fig. 1: Acetate needs to be metabolized to inhibit LHCSR3 accumulation. WT, icl , icl-C and dum11 strains were acclimated for 16 h in LL (15 µmol photons m −2 s −1 ) in HSM; sparged with air (labelled as “air”); sparged with air and supplemented with 10 mM sodium acetate (labelled as “acet”); sparged with air enriched with 5% CO 2 (labelled as “CO 2 ”). After sampling for the LL conditions, light intensity was increased to 600 µmol photons m −2 s −1 (HL); samples were taken 1 h (RNA) or 4 h (protein) after exposure to HL. a , c . Accumulation of LHCSR3 mRNA at the indicated conditions normalized to WT LL ctrl ( n = 3 biological samples, mean ± s.d.). The p-values for the comparisons of acetate and CO 2 conditions to air are based on ANOVA Dunnett’s multiple comparisons test of log10 transformed mRNA data as indicated in the graphs (* P < 0.005, ** P < 0.01, *** P < 0.001, **** P < 0.0001, ns, not significant). Exact p-values can be found at the Source Data file. b , d . Immunoblot analyses of LHCSR3 and ATPB (loading control) under the indicated conditions. Representative datasets of experiments repeated three times. Full size image We evaluated the impact of carbon availability on the photosynthetic properties of cells. The presence of acetate in the medium of WT cells enhanced photosynthetic electron transport (rETR) and strongly suppressed qE (Supplementary Fig. 1 ). In the icl mutant, acetate enhanced the extent of rETR only by ~10% compared with 60% for WT cells. Additionally, acetate caused less pronounced suppression of qE in the icl mutant (by 40%) compared to the level of suppression in WT cells (by 95%); icl-C , behaved similarly to WT cells. As expected, CO 2 enhanced rETR and suppressed qE in WT, icl and icl-C (Supplementary Fig. 1 ). The similarity between the impact of acetate and 5% CO 2 on LHCSR3 expression in WT and icl-C cells (Fig. 1a ) as well as on their photosynthetic properties (Supplementary Fig. 1 ) raised the possibility that both treatments elicited a common mechanism of LHCSR3 control, possibly reflecting a change in the CO 2 concentration within the cell or growth medium. This possibility is plausible based on the finding that acetate metabolism leads to the generation of CO 2 [30] . To investigate whether the generation of CO 2 via acetate metabolism can explain the repression of LHCSR3 transcript and protein levels, we monitored the levels of transcripts from the RHP1 gene in the mutant and WT cells; RHP1 (aka RH1 ) encodes a CO 2 channel shown to be CO 2 responsive and to accumulate in cells grown in a high CO 2 atmosphere [31] . Acetate or 5% CO 2 were introduced to WT and icl mutant cells acclimated in LL and air and the levels of the LHCSR3 and RHP1 transcripts were assayed over a period of 8 h in LL (Fig. 2a, b ). The LHCSR3 transcript accumulation patterns observed agreed with the findings presented in Fig. 1a (LL panel). In WT cells, acetate and CO 2 caused a reduction in LHCSR3 mRNA accumulation over the LL period relative to the control (no acetate, air). Additionally, in the icl mutant, acetate did not affect the accumulation of this transcript while CO 2 efficiently repressed the LHCSR3 transcript level (Fig. 2a ). Under these experimental conditions, acetate levels in the medium decreased in WT cultures but remained unchanged in cultures of the icl mutant (Fig. 2c ). Lastly, RHP1 expression increased in WT and icl mutant cells when the culture was sparged with CO 2 , but only in the WT cells when the cultures were not sparged with CO 2 and only supplemented with acetate, suggesting that acetate metabolism resulted in higher intracellular CO 2 levels (Fig. 2b ). Fig. 2: LHCSR3 inhibition is driven by CO 2 derived from the metabolism of acetate. Experiment at LL: a , b mRNA accumulation of LHCSR3 and RHP1 and c concentration of sodium acetate in the growth medium in WT and icl strains. Cells were acclimated overnight at LL (15 µmol photons m −2 s −1 ) in HSM sparged with air. At t = 0 cells either continued being sparged with air (labelled “air”); or sparged with air and supplemented with 10 mM sodium acetate (labelled “acet”); or sparged with air enriched with 5% CO 2 (labelled “CO 2 ”). The addition of acetate or CO 2 is indicated with a green mark on the x-axis. Samples were taken at t = 0, 1 h, 4 h and 8 h. Experiment at HL: d , e mRNA accumulation of LHCSR3 and RHP1 and f concentration of sodium acetate in the growth medium in WT and icl strains. Cells were acclimated overnight at LL (15 µmol photons m −2 s −1 ) in HSM sparged with air; at t = 0 light intensity was increased to 600 µmol photons m −2 s −1 . At t = 1 h cells either continued being sparged with air (labelled “air”); or sparged with air and supplemented with 10 mM sodium acetate (labelled “acet”); or bubbled with air enriched with 5% CO 2 (labelled “CO 2 ”), always at 600 µmol photons m −2 s −1 . The time of addition of acetate or CO 2 is highlighted in green on the x-axis. Samples were taken at t = 0, 1 h, 2 h, 5 h and 9 h. ( n = 3 biological samples, mean ± s.d.). The p values for the comparisons of acetate and CO 2 conditions to air (LL; t = 1, 4, 8 h, HL; t = 2, 5, 9 h) are based on ANOVA Dunnett’s multiple comparisons test of log10 transformed mRNA data as indicated in the graphs (* P < 0.005, ** P < 0.01, *** P < 0.001, **** P < 0.0001, ns, not significant), following the color-code of the datasets. Exact p-values can be found at the Source Data file. Please note that in some cases the error bars are smaller than the data point symbols. Full size image In another experiment, LL acclimated cells were shifted to HL ( t = 0) and LHCSR3 and RHP1 transcript levels were assayed over a period of 9 h; acetate or high CO 2 were introduced 1 h after the shift to HL (Fig. 2d, e , note the 1 h time point highlighted in green on the x-axis). In agreement with Fig. 1 (HL panel), LHCSR3 transcript accumulation increased by two orders of magnitude after 1 h exposure to HL in both WT and the icl mutant (Fig. 2d ), while RHP1 transcripts rapidly decreased ( Fig. 2e ) , which likely resulted from a reduction in the concentration of intracellular CO 2 as a consequence of enhanced photosynthetic CO 2 fixation in the HL. Introduction of acetate or CO 2 to the cultures caused a rapid reduction in the level of LHCSR3 expression in WT (Fig. 2d ), with the decline much more pronounced with CO 2 supplementation. Supplementation with CO 2 or acetate also caused an increase of RHP1 transcript relative to the control. In contrast, in the icl mutant, the decline in the level of the LHCSR3 transcript and the increase in the level of the RHP1 transcript was the same in cells with and without acetate supplementation, while the effect of CO 2 was similar to that of WT cells (Fig. 2d, e ). Furthermore, WT cells consumed about half of the acetate in the medium over the course of the experiment, while none of the acetate was consumed by the icl mutant (Fig. 2f ). These results strongly suggest that CO 2 inhibits the accumulation of the LHCSR3 transcript and that the decline of LHCSR3 mRNA in WT cells supplemented with acetate is a consequence of the CO 2 released as the acetate is metabolized. The extent of this inhibition by acetate-derived CO 2 appears to depend mostly on the rate of photosynthetic CO 2 fixation (consumption of CO 2 ) because acetate was taken up by WT cells at similar rates under both LL and HL conditions (Fig. 2c, f ). Indeed, under LL conditions, where CO 2 fixation is slow, acetate and CO 2 repressed LHCSR3 to the same extent (Fig. 2a ); under HL conditions, where CO 2 fixation is much faster, the effect of acetate on the LHCSR3 transcript level was much smaller than that of CO 2 , which was continuously provided in excess (5%) via sparging (Fig. 2d ). We also employed constraint-based metabolic modelling to assess in silico whether acetate metabolism in Chlamydomonas leads to an increase in the concentration of intracellular CO 2 under different growth conditions (Supplementary Note 1 , Supplementary Fig. 2 , Supplementary Tables 1 – 3 , Supplementary Data 1 – 3 ). The findings from this approach support the hypothesis that there are changes in the internal CO 2 concentration under autotrophic and mixotrophic growth conditions at different light intensities. These predicted changes in internal CO 2 levels under the different conditions for the WT and mutant cells are congruent with the levels of accumulation of LHCSR3 transcripts that were measured. 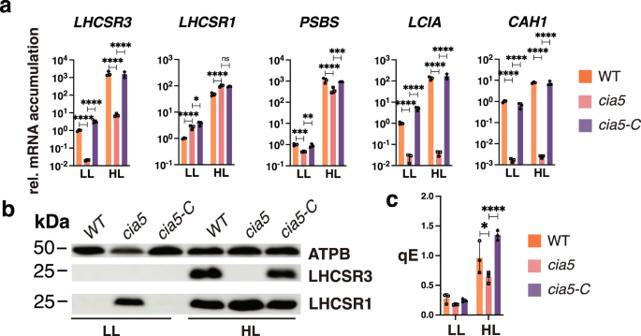Fig. 3: Cross-talk of responses to HL and low-CO2. aCC-125 WT,cia5andcia5-c strains were acclimated for 16 h in LL (15 µmol photons m−2s−1) in HSM bubbled with air (labelled as “LL”); after sampling for the LL conditions, light intensity was increased to 600 µmol photons m−2s−1(HL); samples were taken after 1 h (RNA) and 4 h (protein and photosynthesis measurements). Accumulation of mRNA of genes at the indicated conditions were normalized to WT LL ctrl. (n= 3 biological samples, mean ± s.d.). The p-values for the comparisons of WT withcia5andcia5withcia5-Care based on ANOVA Dunnett’s multiple comparisons test of log10 transformed mRNA data as indicated in the graphs.bImmunoblot analyses of LHCSR3, LHCSR1 and ATPB (loading control) under the indicated conditions; PSBS was non-detectable at these experimental conditions. Representative dataset of experiment repeated three times.cqE of WT,cia5andcia5-Cunder LL and HL conditions (n= 3 biological samples, mean ± s.d.). The statistical analyses (two-way ANOVA Tukey’s multiple comparison test) are shown in the graph. Exact p-values can be found at the Source Data file. Raw fluorescence and NPQ curves can be seen in Supplementary Fig.4. CIA5 links HL and low CO 2 responses The responses to HL and low CO 2 have been traditionally studied separately, despite several lines of evidence suggesting that they are integrated [26] , [27] , [32] . To elucidate the molecular connection between photoprotection and CCM, we analyzed mRNA accumulation of twelve genes implicated as functionally involved in the CCM, previously shown to be strongly expressed under low CO 2 conditions [33] , [34] and/or to be under the control of CIA5 [26] . Specifically, we analysed twelve CCM-related genes encoding LOW-CO 2 -INDUCIBLE PROTEIN B (LCIB) and E (LCIE), involved in CO 2 uptake; HIGH-LIGHT ACTIVATED 3 (HLA3), LOW CO 2 -INDUCED 1 (LCI1), CHLOROPLAST CARRIER PROTEIN 1 (CCP1), CCP2, LCIA, BESTROPHINE-LIKE PROTEIN 1 (BST1), acting as Ci transporters; carbonic anhydrases CAH1, CAH3, CAH4; the nuclear regulator LOW-CO 2 -STRESS RESPONSE 1 (LCR1). When LL-acclimated, air-sparged WT, icl and icl-C strains were exposed to HL (experiment described in Fig. 1 ) a marked increase (5 to 600-fold) in CCM transcript levels was observed in WT cells (Supplementary Fig. 3 ), in accordance with recent studies; [28] , [32] this increase was strongly suppressed by CO 2 and to a lesser extent by acetate, which did not affect CCM gene expression in the icl mutant (Supplementary Fig. 3 ). This pattern of mRNA accumulation was essentially identical to that of LHCSR3 (Fig. 1a ), highlighting the tight connection between HL and low-CO 2 responses in Chlamydomonas . The CO 2 -mediated repression was more pronounced for most of the CCM genes relative to LHCSR3 (Fig. 1a, c , Supplementary Fig. 3 ). CIA5 has been shown to regulate the accumulation of transcripts from both the CCM genes [26] , [27] and LHCSR3 [28] . To obtain a comprehensive view of the photoprotection capacity of the cia5 mutant, air-sparged WT and cia5 cells grown in LL were shifted to HL, and the transcript and protein levels from the qE effector genes were monitored. Remarkably, a lack of CIA5 resulted in much lower accumulation of LHCSR3 mRNA than in WT cells; 50 times lower at LL and over 200 times lower at HL. This phenotype was fully reversed by ectopic expression of the WT CIA5 gene (Fig. 3a ). PSBS also showed a significant CIA5-dependent control at the mRNA level, although at a smaller extent (Fig. 3a ). The cia5 mutant accumulated slightly more LHCSR1 mRNA in both LL and HL (~2 fold), however, this phenotype was not restored in the complemented cia5-C strain (Fig. 3a ); we conclude that LHCSR1 mRNA accumulation is CIA5-independent. We also quantified the accumulation of mRNAs of CAH1 and LCIA , which are known to be strongly dependent on CIA5 [27] , [35] . As expected, the cia5 mutant cells failed to activate either of those genes in HL while their activation was fully restored in the complemented cia5-C strain (Fig. 3a ). Fig. 3: Cross-talk of responses to HL and low-CO 2 . a CC-125 WT, cia5 and cia5 -c strains were acclimated for 16 h in LL (15 µmol photons m −2 s −1 ) in HSM bubbled with air (labelled as “LL”); after sampling for the LL conditions, light intensity was increased to 600 µmol photons m −2 s −1 (HL); samples were taken after 1 h (RNA) and 4 h (protein and photosynthesis measurements). Accumulation of mRNA of genes at the indicated conditions were normalized to WT LL ctrl. ( n = 3 biological samples, mean ± s.d.). The p-values for the comparisons of WT with cia5 and cia5 with cia5-C are based on ANOVA Dunnett’s multiple comparisons test of log10 transformed mRNA data as indicated in the graphs. b Immunoblot analyses of LHCSR3, LHCSR1 and ATPB (loading control) under the indicated conditions; PSBS was non-detectable at these experimental conditions. Representative dataset of experiment repeated three times. c qE of WT, cia5 and cia5-C under LL and HL conditions ( n = 3 biological samples, mean ± s.d.). The statistical analyses (two-way ANOVA Tukey’s multiple comparison test) are shown in the graph. Exact p-values can be found at the Source Data file. Raw fluorescence and NPQ curves can be seen in Supplementary Fig. 4 . Full size image At the protein level, no LHCSR3 protein was detected in the cia5 mutant in either LL or HL ( Fig. 3b ). We were unable to immunologically detect the PSBS protein under these experimental conditions, in agreement with previous findings showing that PSBS protein accumulation is highly transient in cell cultures bubbled with air [6] . Importantly, the LHCSR1 protein accumulated to high levels in the mutant under both LL (conditions in which no protein is apparent in the WT) and HL conditions; this phenotype was fully reversed by ectopic expression of the WT CIA5 gene (Fig. 3b ). This result suggests that CIA5 acts as a suppressor of LHCSR1 translation (and/or decreases protein stability) in both LL and HL. Our data additionally suggest that accumulation of LHCSR1 protein occurs through a compensatory, CIA5-controlled posttranscriptional mechanism that provides photoprotection under conditions in which the cells have almost no LHCSR3 protein (compare LHCSR1 and LHCSR3 immunoblots in Fig. 3b ). Supporting this idea, the qE levels in cia5 , although lower than WT and cia5-C (Fig. 3c and Supplementary Fig. 4 ), they were unexpectedly high considering the absence of LHCSR3 protein (Fig. 3b ); we attribute this result to overaccumulation of LHCSR1 in this mutant (Fig. 3b ). Together, our results demonstrate a key role of CIA5 in regulating photoprotection, activating LHCSR3 and to a lesser extent PSBS transcription and suppressing LHCSR1 protein accumulation. CIA5 and CO 2 availability regulate LHCSR1 protein stability The high levels of accumulation of LHCSR1 protein in the cia5 mutant (Fig. 3b ) suggest that CO 2 availability could be the key determinant for LHCSR1 protein accumulation, as CIA5 is not functional under high CO 2 levels [15] , [16] , [17] . Given the novelty of this finding, we decided to perform additional experiments to provide more details concerning LHCSR1 regulation. LL-acclimated WT cells sparged with air were exposed to HL sparged with air or 5% CO 2 and the mRNA and protein levels were quantified over a 25-h period. Upon initial exposure to HL, LHCSR1 mRNA rapidly increased (2 orders of magnitude in 1 h) and then decreased to the initial level (between 4 and 8 h), in agreement with a previous report [36] , in the presence or absence of high CO 2 (Fig. 4a ). In contrast, the presence of high CO 2 sustained high levels of LHCSR1 protein over the 25-h incubation period relative to cultures sparged with air (Fig. 4b ). These results suggest that elevated CO 2 either promotes translation of LHCSR1 mRNA or is involved in stabilizing the protein once it is synthesized. This contrasts with the behaviour of LHCSR3 for which there was a strong correlation between the level of mRNA and protein (the RNA was 3 orders of magnitude lower in 5% CO 2 and the protein was no longer detected) (Fig. 4 ). The kinetics of PSBS transcript accumulation in HL very much resembled those of LHCSR1 , with CO 2 not having a strong impact on transcript accumulation (Fig. 4a ). PSBS protein accumulation was not detectable under the experimental conditions used. Taken together, our data demonstrate the critical importance of CIA5 and CO 2 in regulating the different qE effectors, mainly LHCSR3 and less strongly PSBS at the transcript level, and LHCSR1 at the protein level. Fig. 4: Kinetic resolution of photoprotective gene and protein expression at different light and CO 2 availabilities. Cells were acclimated overnight at LL (15 µmol photons m −2 s −1 ) bubbled with air (labelled “air”). At t = 0 the light intensity was raised to 600 µmol photons m −2 s −1 under air bubbling or bubbling with 5% CO 2 and mRNA and protein were followed for 25 h. a LHCSR1, LHCSR3 and PSBS mRNA accumulation. ( n = 3 biological samples, mean ± s.d.). The p-values for the comparisons of CO 2 conditions to air for t = 1, 4, 8, 24 and 25 h are based on two-way ANOVA Šídák’s multiple comparisons test of log10 transformed mRNA data as indicated in the graphs (* P < 0.005, ** P < 0.01, *** P < 0.001, **** P < 0.0001, ns, not significant). Exact p-values can be found at the Source Data file. b Immunoblot analyses of LHCSR1, LHCSR3 and ATPB (loading control). Representative dataset of experiment repeated three times. Full size image Intracellular CO 2 levels regulate photoprotective and CCM gene expression in the absence of light To de-convolute the light and CO 2 signals regulating LHCSR3 , we exposed the cells to different light intensities and CO 2 concentrations (Supplementary Fig. 5 ). High CO 2 levels completely abolished the accumulation of LHCSR3 protein at all light intensities, in accord with the results of Fig. 1b, d and Fig. 4b . On the contrary, low CO 2 levels led to very high accumulation of LHCSR3 protein at 150 and 300 µmol photons m −2 s −1 . Under low CO 2 , LHCSR3 protein was also detectable even at the very low light intensity of 10 µmol photons m −2 s −1 ( Supplementary Fig. 5 ), as previously demonstrated [6] . Prompted by this result, we tested whether changes in CO 2 levels could activate transcription of LHCSR3 in complete darkness. We shifted air-sparged cells to sparging with CO 2 -free air (Very low CO2; VLCO 2 ) in complete darkness and to our surprise, we observed that despite the absence of light, that a drop in CO 2 availability was sufficient to trigger LHCSR3 mRNA accumulation by ~ 700-fold (Fig. 5a ), with an increase in accumulation of the protein by 3-fold (Fig. 5b, c ; compare WT air with WT VLCO 2 ). In addition, when HL was combined with VLCO 2 , which is expected to result in an even greater reduction in the intracellular CO 2 concentration, the levels of LHCSR3 mRNA and protein further increased, reaching levels of ~4500-fold (mRNA) and 21-fold (protein) compared to air dark conditions (Fig. 5a-c ). Interestingly, this light-independent regulation of mRNA accumulation was under the control of CIA5 as the accumulation of LHCSR3 transcripts was abolished in the cia5 mutant (Fig. 5a ) and a full reversal of these phenotypes (gene expression and protein levels) was observed in the cia5-C strain (Fig. 5a, b ). We also observed significant LHCSR3 transcript accumulation in the cia5 mutant when cells were shifted from dark-air to HL-VLCO 2 , which was, however, 9-fold lower compared to the WT (Fig. 5a ), and that was rescued to WT-levels in the cia5-C complemented line. This CIA5-independent regulation of mRNA in the presence of light could account for the contribution of light signaling in LHCSR3 gene expression, possibly via phototropin [10] or via the generation of reactive oxygen species [28] . Fig. 5: Low CO 2 levels can trigger qE and CCM genes in the absence of light. WT, cia5 and cia5-C cells were bubbled with air overnight in darkness; next day air bubbling was either maintained or replaced by CO 2 -limited-air bubbling in the darkness or in the presence of 600 µmol photons m −2 s −1 light. Sampling was performed after 1 h (RNA) or 4 h (protein). a mRNA accumulation of LHCSR3.1 (qE gene) and CAH4, LCIA, LCI1 (CCM genes) in WT, cia5 and cia5-C . Data were normalized to WT air dark; ( n = 3 biological samples, mean ± s.d.). The p-values for the comparisons of WT with cia5 and cia5 with cia5-C are based on ANOVA Dunnett’s multiple comparisons test of log10 transformed mRNA data as indicated in the graphs (* P < 0.005, ** P < 0.01, *** P < 0.001, **** P < 0.0001, ns, not significant). Exact p-values can be found at the Source Data file. b Immunoblot analyses of LHCSR3 and ATPB (loading control) under the indicated conditions. Representative dataset of experiment repeated three times. c Immunoblot analyses of LHCSR3 and ATPB (loading control) of WT samples presented in b . Above the immunoblot shown are the amount of protein loaded per lane and the quantification of LHCSR3 protein accumulation (calculated as LHCSR3 /ATPB ratio) normalized to the air dark conditions. Representative dataset of experiment repeated three times. Full size image We could observe that LHCSR1 transcripts were also induced in the dark (shift from dark-air to dark-VLCO 2 ), but this induction was very low (7-fold) and appeared to be CIA5 independent (Supplementary Fig. 6a ). At the protein level however, LHCSR1 over-accumulated in the cia5 mutant under all conditions tested (Supplementary Fig. 6b ), confirming our previous findings (Fig. 3b ) . PSBS also showed a CIA5-dependent dark induction of transcripts (shift from dark-air to dark-VLCO 2 ), although this induction was low (5-fold); complementation with the CIA5 gene ( cia5-C strain) did not rescue the phenotype in dark-air conditions and only partially rescued it under dark-VLCO 2 (Supplementary Fig. 6a, b ). Both mRNA and protein accumulation of PSBS accumulated in a CIA5-dependent manner when cells were shifted from dark-air to HL-VLCO 2 (Supplementary Fig. 6a, b ); under these conditions the phenotypes were fully reversed in the cia5-C strain. This CIA5-dependent regulation of PSBS can most likely explain previously reported findings that PSBS protein accumulation was responsive to CO 2 abundance, with its accumulation reaching maximum levels under low CO 2 and HL conditions [6] . We also measured CCM-related gene expression in the dark. As shown in Fig. 5a and Supplementary Fig. 6a , high levels of CCM-related transcripts were observed in the dark when the cells experienced VLCO 2 conditions (compare “dark air” with “dark VLCO 2 ”). The combination of HL and VLCO 2 conditions, either elicited very small (less than two-fold) or no additional increase (compare “HL VLCO 2 ” to “dark VLCO 2 ”) in their level of the mRNA accumulation (Fig. 5a and Supplementary Fig. 6a ). As expected CIA5 was critical for expression of the CCM genes under all conditions tested ( Fig. 5a and Supplementary Fig. 6a ). Our data points out that the LHCSR1 protein overaccumulation in cia5 was fully reversed only when cia5-C cells were pre-acclimated in the light (Fig. 3b ); when pre-acclimation took place in the dark the phenotype was only partially rescued (Supplementary Fig. 6b ). The same is true for the mRNA accumulation of PSBS (compare LL; Fig. 3a with air-dark; Supplementary Fig. 6a ), CAH1 (compare LL; Fig. 3a with air-dark; Supplementary Fig. 6a ), LCIA (compare LL; Fig. 3a with air-dark; Fig. 5a ), while in the case of LHCSR3 a full reversal of the CIA5-dependent phenotype was seen no matter what pre-acclimation strategy was followed (Figs. 3a, b and 5a, b ). A plausible explanation for these results is the differential accumulation of CIA5 protein in the different acclimation regimes due to the promoter used. In line with this explanation, CIA5 expression in cia5-C is driven by the light-inducible promoter of the PSAD gene, and, as a result, less CIA5 protein accumulated in the dark-acclimated cia5-C compared to the LL-acclimated (Supplementary Fig. 7a ). This in turn affects the relative abundance of CIA5 available for binding with its target molecules (DNA binding sites or CIA5-interacting proteins), ultimately affecting the reversal of the CIA5-related phenotypes. Overall, these data challenge the view concerning the regulation of photoprotection and CCM and bring CO 2 to the forefront as a crucial signal controlling LHCSR3 and CCM-related genes induction in the absence of light. Link between photosynthetic electron transfer and CO 2 intracellular concentration Our finding that LHCSR3 is regulated by light-independent CO 2 availability has guided us in revising the way in which we view the impact of photosynthetic electron transfer ( PET) on LHCSR3 accumulation; i.e. inhibition of LHCSR3 accumulation in photosynthetic mutants or WT cells treated with photosynthetic inhibitors [10] , [11] . We propose that enhanced PET, occurring under HL conditions, facilitates CO 2 fixation, draws down the intracellular CO 2 concentration and induces LHCSR3 transcription. In contrast, when PET is impaired, intracellular CO 2 levels increase, thus promoting LHCSR3 transcript inhibition. In accordance, there is a marked increase of CO 2 in cultures treated with DCMU, an inhibitor of photosystem II [37] , measured either as dissolved CO 2 in the culture medium [30] , or as CO 2 in the air stream coming from the headspace of the column bioreactor (Fig. 6a ). In order to test our hypothesis, we analyzed the combined effect of DCMU and CO 2 on the accumulation of mRNA from the LHCSR3 and two CCM genes in WT cultures shaken without or with VLCO 2 sparging. In accord with previous reports [10] , [38] , DCMU completely blocked the HL elicited accumulation of LHCSR3 mRNA; LHCSR3 mRNA after 1 h exposure to HL diminished to ten times lower levels than the initial LL levels (shown as dotted line in graph) (Fig. 6b ), which most likely reflects the degradation of the transcripts following inactivation of the gene after the addition of DCMU. Previous work has shown that LHCSR3 transcripts are rapidly lost once the gene becomes inactive [10] which has also been observed for the CAH4 transcript [39] . However, when the cultures were sparged with VLCO 2 air, which would result in the maintenance of a continuous VLCO 2 concentration in the cultures, a large part of the DCMU elicited inhibition was relieved (Fig. 6b ), supporting the idea that light primarily impacts LHCSR3 transcript levels by altering CO 2 consumption and the intracellular (and/or extracellular) CO 2 concentration. In contrast to LHCSR3 , sparging with VLCO 2 only partly relieved the suppression of transcript accumulation for the CCM genes in the presence of DCMU (Fig. 6b ). This difference may reflect the fact that CCM gene expression is solely regulated by CO 2 via CIA5 (Fig. 5a ) and that sparging with VLCO 2 in the presence of DCMU does not reduce the CO 2 levels enough to attain full gene activation. It is also possible that longer incubation time with VLCO 2 would have relieved a larger part of the DCMU-elicited inhibition of CCM genes (Fig. 6b ) as implied by the slow kinetics of CAH4/5 mRNA accumulation when cells are shifted from 5% CO 2 to air [39] . Fig. 6: Photosynthetic electron transfer draws down the intracellular CO 2 concentration, relieving inhibition of LHCSR3 transcription. a CO 2 concentration measured in the air stream coming out of the headspace of a column filled with 50 mL of HSM, sparged with air under HL. The two arrows in the graph indicate the addition of cells or DCMU. b WT cells were acclimated to LL HSM overnight shaken in flasks; the next day they were exposed to 300 µmol photons m −2 s −1 light in the presence or absence of 40 µM DCMU, shaken in flasks without or with sparging with VLCO 2 . Samples were taken after 1 h. Presented are mRNA accumulation of LHCSR3 , CAH4 , LCIA . Data were normalized to LL (shown as dotted line in graph); n = 2 biological samples. Full size image In this work, we presented findings that advance our understanding of integration between CO 2 - and light-dependent signaling in Chlamydomonas . We propose that the intracellular level of CO 2 , defined by the equilibrium between light-driven CO 2 fixation in chloroplasts and the generation of CO 2 by mitochondrial metabolism (e.g. acetate assimilation), is a key regulator of two major processes in photosynthetic organisms: the CCM and photoprotection (Fig. 7 ). Fig. 7: CO 2 - and light-dependent signals converge to regulate photoprotection and CCM in Chlamydomonas. The intracellular levels of CO 2 , defined by the equilibrium between CO 2 fixation in chloroplasts and the generation of CO 2 by mitochondrial metabolism (e.g. acetate assimilation) is the key determinant of the regulation of gene expression controlling two major processes of photosynthetic organisms: CCM and photoprotection. Changes in light availability have a direct impact on intracellular CO 2 levels; exposure to HL increases CO 2 fixation rates leading to depletion of CO 2 and to activation of not only photoprotection- but also CCM-related genes. Conversely, depletion of CO 2 is sufficient to drive high expression levels of CCM genes and LHCSR3 even in complete darkness (indicated by the black arrows). High CO 2 levels, either exogenously supplied by sparging or metabolically produced via acetate metabolism or by inhibiting photosynthetic electron flow using DCMU, repress LHCSR3 and CCM genes while at the same time they stabilize LHCSR1 protein levels. The close interconnection of photoprotection and CCM is further corroborated by the fact that CIA5, the regulator of expression of genes associated with the CCM, also exerts control over LHCSR3 and to a lesser extent over PSBS mRNA levels and acts as repressor of LHCSR1 protein accumulation. Independent of CIA5, light strongly impacts expression of all of these photoprotective genes (yellow arrows). This impact can be the consequence of both photoperception (e.g. phototropin) and the production of reactive oxygen species. Full size image To better understand the role of CO 2 in regulating photoprotection and its integration with light, we designed experiments to separate the effects of the two signals (Figs. 5 – 7 ); we reduced the concentration of CO 2 in the microalgae medium by sparging it with VLCO 2 in complete darkness. This abrupt change in CO 2 levels experienced by the cultures in the dark may be considered a condition only encountered in the laboratory. However, in certain ecological niches, such as soil or catchments with elevated levels of organic matter [33] , Chlamydomonas would encounter changes in the levels of CO 2 that would be dependent on the microbes and the ratio between respiration and photosynthesis in the environment. Our experimental setup allowed us to observe a strong increase of LHCSR3 transcript levels when cells were shifted from air-CO 2 to VLCO 2 levels in the dark (Fig. 5 ), a very surprising result as the accumulation of LHCSR3 mRNA was considered so far to be strictly light-dependent [5] , [11] , [38] . Moreover, with this strategy we can disentangle light from CO 2 signalling effects; while dark induction of LHCSR3 under CO 2 -depletion was completely dependent on CIA5, light could still strongly impact expression of all photoprotective genes in the cia5 mutant, which was not the case for CCM gene expression that was completely abolished in the light or dark in the absence of CIA5 (Fig. 5 and Supplementary Fig. 6 ). This impact of light on qE gene expression may be the consequence of photoperception (e.g. PHOT1) [10] , but also the generation of light-dependent signals such as reactive oxygen species [28] . Furthermore, a CIA5-independent regulation (also observed in Fig. 3a ) explains LHCSR3 induction in high CO 2 -acclimated WT cells (cells in which CIA5 is not functional [15] , [16] , [17] ) as they transition from LL to HL (Fig. 1a ), which was not observed for CCM genes tested under identical conditions (Supplementary Fig. 3 ); it also explains why the CO 2 -mediated repression was more pronounced for most of the CCM genes relative to LHCSR3 (Fig. 1a, c , Supplementary Fig. 3 ). CO 2 and CIA5 appear to be of paramount importance in signal integration and transduction, regulating expression of both photoprotection and CCM genes. For instance, CO 2 represses the UV-B elicited, UVR8-mediated expression of LHCSR3 , and CIA5 is absolutely required for this expression [28] . Moreover, our results have shown that high CO 2 levels or the absence of CIA5 have a severe impact on LHCSR3 gene expression and, although HL can still induce LHCSR3 transcription, no protein is detected (Figs. 1 , 3 and 5 ). Besides transcriptionally controlling LHCSR3 , CIA5 post-transcriptionally controls LHCSR1. Our view on LHCSR1 regulation by light and CIA5 is as follows: under LL conditions, LHCSR1 protein accumulates in cia5 while it is non-detectable in WT and cia5-C (Fig. 3b ), suggesting that CIA5 suppresses LHCSR1 protein accumulation. Exposure to HL triggers a CIA5-independent LHCSR1 mRNA accumulation (Fig. 3a ), possibly driven by reactive species, previously shown to favor LHCSR1 mRNA accumulation [40] . As a result, LHCSR1 protein accumulates in WT and cia5-C in HL, despite the fact that suppression of LHCSR1 protein by CIA5 still occurs; indeed, LHCSR1 accumulates to higher levels in the cia5 mutant as compared to WT and cia5-C under HL conditions (Fig. 3b ). In line with the above observations in the cia5 mutant, high levels of LHCSR1 protein accumulate in WT under high CO 2 , conditions that inactivate CIA5 (Fig. 4b ). Put together, our findings unveil a multilevel role of CIA5 in regulating qE; inactivation of CIA5 in high CO 2 or by eliminating the CIA5 gene blocks LHCSR3 transcript accumulation, while it promotes LHCSR1 protein accumulation (Figs. 3 , 4 ). Further investigation will be required to explain how a single nuclear factor, CIA5, can control cellular processes happening in different cellular compartments; transcription in the nucleus and translation in the cytosol. Our results provide an interpretation of the findings that PET is required for LHCSR3 accumulation [11] , activation of the CCM and expression of CCM genes [41] . We propose that CO 2 , either provided directly or indirectly through metabolic generation, represents a critical link between PET and transcriptional regulation of LHCSR3 and the CCM genes (Fig. 6 ). Photosynthesis draws down cellular CO 2 levels, and therefore, blocking photosynthesis with DCMU leads to the accumulation of CO 2 (Fig. 6a ) which elicits LHCSR3 repression, while sparging DCMU-treated cells with VLCO 2 almost fully derepresses LHCSR3 (and partially CCM) expression (Fig. 6b ). DCMU also upregulates genes of the leucine degradation pathway [42] leading to the generation of acetoacetate and acetyl-CoA, which can lead to oxidative CO 2 production. Whether leucine itself has a regulatory role or CO 2 is the key regulator deserves further attention. It is tempting to propose that CO 2 is a retrograde signal that readily diffuses through the cell and impacts nuclear gene expression, which would integrate both mitochondrial and chloroplastic metabolic activities. The way in which Chlamydomonas senses CO 2 is not clear. Our data, i.e. accumulation of LHCSR3 and CCM genes in the dark, exclude the possibility that a metabolite produced by photorespiration plays a major signalling role, as previously proposed [43] . CO 2 itself might also serve as the metabolite being recognized by a putative sensor that could be controlled by carbamylation, a CO 2 -mediated post-translational modification that regulates, among others, the activation of Rubisco [44] . Furthermore, the large number of adenosine and guanylyl cyclases in Chlamydomonas [45] suggests that cyclic nucleotides play an important role in controlling various processes in this alga; these metabolites have been shown to be involved in mating [46] , regulation of flagellar beating and phototaxis [47] , [48] , [49] , in regulating inorganic nitrogen assimilation [50] and in restoring LHCSR3 accumulation in the absence of phototropin [10] . Cyclases have been shown to act as CO 2 sensors (as bicarbonate) in mammalian cells [51] , making it plausible that they can also serve as sensors in Chlamydomonas . As cyclic nucleotide signalling and calcium are tightly linked [51] , we anticipate an important role for calcium in CO 2 sensing; calcium signalling has already been shown to be involved in the regulation of both LHCSR3 and CCM genes [11] , [52] . Overall, our work shows that the intracellular CO 2 level is the main factor in regulating CCM genes and LHCSR3 in Chlamydomonas (Fig. 7 ). Exposure to HL increases the CO 2 fixation rate which causes a drop in intracellular CO 2 which, in turn, actives both photoprotection- and CCM-related genes. Depletion of CO 2 is sufficient to drive high expression levels of CCM genes and LHCSR3 even in complete darkness. On the other hand, high CO 2 levels, either generated through enhanced respiratory activity or impaired photosynthetic electron transport, repress LHCSR3 and CCM genes while at the same time stabilizing the LHCSR1 protein, which likely acts as a backup photoprotection protein under conditions where LHCSR3 is not expressed. Furthermore, our data reveals a closer interconnection of photoprotection and CCM as CIA5, the CCM master regulator, also exerts control over LHCSR3 and to a lesser extent over PSBS mRNA levels, while repressing LHCSR1 protein accumulation. Our findings highlight the need to develop an integrated approach that examines the role of CO 2 and light, not only as substrates of photosynthetic CO 2 fixation, but also as signals regulating photoprotection, CCM, and at a wider context genome-wide gene expression. Chemicals DCMU (3-(3,4-dichlorophenyl)−1,1-dimethylurea) was purchased from Sigma. Stock solutions of DCMU were prepared in ethanol (40 mM). Strains and conditions Chlamydomonas strains were grown under 20 µmol photons m −2 s −1 in Tris-acetate-phosphate (TAP) medium [53] at 23 °C in Erlenmeyer flasks shaken at 125 rpm. For all experiments cells were transferred to Sueoka’s High Salt medium [54] supplemented when needed with 10 mM sodium acetate, at 2 million cells mL −1 in 80 mL capacity columns, unless otherwise stated, sparged with air, air enriched with 5% CO 2 , or very low CO 2 air (VLCO 2 ; generated by passing the air through soda lime) and exposed to light intensities as described in the text and figure legends. Chlamydomonas strain 137c mt+ was used as WT. The icl (defective in ICL1 ; gene ID: Cre06.g282800) , icl-C ( icl strain complemented with the WT ICL gene), dum11 (defective in defective in ubiquinol cytochrome c oxidoreductase of the respiratory complex III; geneID: CreMt.g000300) and cia5 (defective in CIA5 , aka CCM1; geneID: Cre02.g096300; Chlamydomonas Resource Centre strain CC-2702) mutants were previously generated [15] , [21] , [29] . 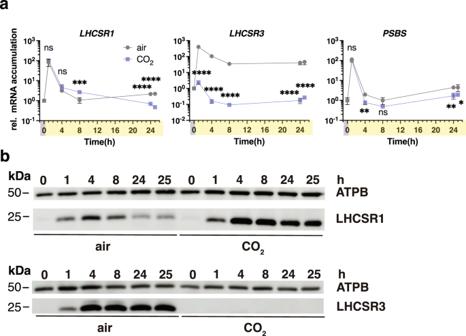Fig. 4: Kinetic resolution of photoprotective gene and protein expression at different light and CO2availabilities. Cells were acclimated overnight at LL (15 µmol photons m−2s−1) bubbled with air (labelled “air”). At t = 0 the light intensity was raised to 600 µmol photons m−2s−1under air bubbling or bubbling with 5% CO2and mRNA and protein were followed for 25 h.aLHCSR1, LHCSR3andPSBSmRNA accumulation. (n= 3 biological samples, mean ± s.d.). The p-values for the comparisons of CO2conditions to air for t = 1, 4, 8, 24 and 25 h are based on two-way ANOVA Šídák’s multiple comparisons test of log10 transformed mRNA data as indicated in the graphs (*P< 0.005, **P< 0.01, ***P< 0.001, ****P< 0.0001, ns, not significant). Exact p-values can be found at the Source Data file.bImmunoblot analyses of LHCSR1, LHCSR3 and ATPB (loading control). Representative dataset of experiment repeated three times. For complementation of cia5 , a 3.5-kbp genomic DNA fragment from CC-125 containing the CIA5 coding region was amplified by PCR using Platinum™ SuperFi™ DNA Polymerase (Thermo Fisher Scientific) and primers gib-cia5-fw and gib-cia5-rev (Supplementary Table 4 ), gel purified and cloned into pLM005 [55] by Gibson assembly [56] for expression under control of the PSAD promoter. Junctions and insertion were sequenced, and constructs were linearized by EcoRV before transformation into cia5 . Eleven ng/kb of linearized plasmid [55] mixed with 400 μL of 1.0 × 10 7 cells mL −1 were electroporated in a volume of 120 mL in a 2-mm-gap electro cuvette using a NEPA21 square-pulse electroporator (NEPAGENE, Japan). The electroporation parameters were set as follows: Poring Pulse (300 V; 8 ms length; 50 ms interval; one pulse; 40% decay rate; + Polarity), Transfer Pulse (20 V; 50 ms length; 50 ms interval; five pulses; 40% decay rate; +/- Polarity). Transformants were plated onto solid agar medium containing 10 μg/ml paromomycin and screened for fluorescence using a Tecan fluorescence microplate reader (Tecan Group Ltd., Switzerland). Parameters used were as follows: YFP (excitation 515/12 nm and emission 550/12 nm) and chlorophyll (excitation 440/9 nm and 680/20 nm). Transformants showing a high YFP/chlorophyll ratio were further analyzed by immunoblotting using anti-FLAG antibodies (Supplementary Fig. 7b ). Among the transformants analyzed the cia5-C-a1 ( cia5-C throughout the text) was retained for further analyses in the present study, after verifying that it grows similarly with the WT under phototrophic conditions on agar (Supplementary Fig. 7c ). Unless otherwise stated, LL conditions corresponded to 20 µmol photons m −2 s −1 while HL conditions corresponded to 600 µmol photons m −2 s −1 of white light (Neptune L.E.D., France; see Supplementary Fig. 8 for light spectrum). All experiments were repeated three times to examine reproducibility, unless otherwise stated. Light acclimation experiments Cells were acclimated overnight in High Salt Medium (HSM) in LL sparged with air, in the presence or absence of acetate, or sparged with 5% CO 2 . Following this acclimation period, cells were transferred from LL to HL, with all other conditions identical to those of the acclimation period. Samples were collected after 1 h for RNA analyses and after 4 h for protein analysis and measurements of photosynthetic activity. Fluorescence-based measurements Fluorescence-based photosynthetic parameters were measured with a pulse modulated amplitude fluorimeter (MAXI-IMAGING-PAM, HeinzWaltz GmbH, Germany). Prior to the onset of the measurements, cells were acclimated to darkness for 15 min. Chlorophyll fluorescence was recorded under different intensities of actinic light; starting with measurements in the dark (indicated as D below the x-axis of the graphs), followed by measurements at 21 μmol photons m −2 s −1 (indicated as L1 below the x-axis of the graphs) and 336 μmol photons m −2 s −1 (indicated as L2 below the x-axis of the graphs) and finishing with measurements of fluorescence relaxation in the dark. The calculations of the different photosynthetic parameter was performed based on [57] as follows: The relative photosynthetic electron transfer rate (rETR) was calculated as ( F m′ − F )/ F m ′ × I; F and F m′ are the fluorescence yield in steady state light and after a saturating pulse in the actinic light, respectively; I is the light irradiance in μmol photons m −2 s −1 ; NPQ was calculated as ( F m − F m′)/ F m′; F m is the maximal fluorescence yield in dark-adapted cells; the effective photochemical quantum yield of photosystem II was calculated as Y(II) = (Fm’-F)/Fm’; qE was estimated as the fraction of NPQ that is rapidly inducible in the light and reversible in the dark. mRNA quantification Total RNA was extracted using the RNeasy Mini Kit (Qiagen) and treated with the RNase-Free DNase Set (Qiagen). 1 µg total RNA was reverse transcribed with oligo dT using Sensifast cDNA Synthesis kit (Meridian Bioscience, USA). qPCR reactions were performed and quantitated in a Bio-Rad CFX96 system using SsoAdvanced Universal SYBR Green Supermix (BioRad). The primers (0.3 µM) used for qPCR are listed in Supplementary Table 4 . A gene encoding G protein subunit-like protein (GBLP) [58] was used as the endogenous control, and relative expression values relative to GBLP were calculated from three biological replicates, each of which contained three technical replicates. CO 2 measurements CO 2 concentration was measured in the air stream coming from the headspace of a HSM or culture-containing column using the CO 2 Probe GMP251 connected to the MI70 data logger from Vaisala (Vantaa, Finland). Immunoblotting Protein samples of whole cell extracts (0.5 µg chlorophyll or 10 µg protein) were loaded on 4-20% SDS-PAGE gels (Mini-PROTEAN TGX Precast Protein Gels, Bio-Rad) and blotted onto nitrocellulose membranes. Antisera against LHCSR1 (AS14 2819, 1:15000 dilution), LHCSR3 (AS14 2766, 1:15000 dilution), ATPB (AS05 085, 1:15000 dilution) were from Agrisera (Vännäs, Sweden); previously described was antisera against C. reinhardtii PSBS [6] (used at a dilution of 1:1000). ATPB was used as a loading control. An antirabbit horseradish peroxidase-conjugated antiserum was used for detection at 1:10000 dilution. Mouse monoclonal antibody against FLAG was purchased from Sigma-Aldrich (F3165, St. Louis, MO, USA) and was used at a dilution of 1:15000. An anti-mouse horseradish peroxidase-conjugated antiserum (Jackson Immuno Research Europe LTD) was used as a secondary antibody for 3xFLAG immunoblotting (1:10000 dilution). The blots were developed with ECL detection reagent, and images of the blots were obtained using a CCD imager (ChemiDoc MP System, Bio-Rad). For the densitometric quantification, data were normalized with ATPB. Statistical analyses Statistical methods were not used to predetermine the sample size. The experiments were not randomized, and the investigators were not blinded to allocation during experimental procedures and data assessment. All statistical tests were performed using the computing environment Prism 9 (Graphpad Software, LLC), at a significance level of 0.05. In order to conform mRNA accumulation data to the distributional assumptions of Analysis of Variance (ANOVA), i.e. the residuals should be normally distributed and variances should be equal among groups, two-way ANOVA was performed with log-transformed data Y = logX where X is mRNA accumulation [59] . 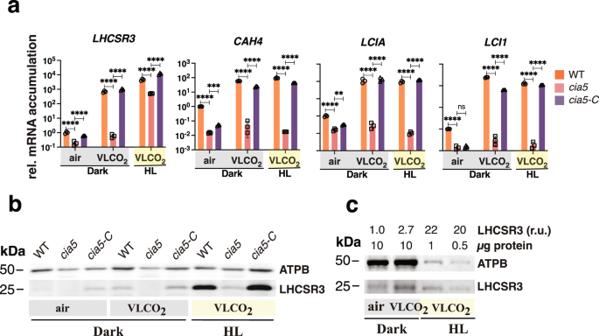Fig. 5: Low CO2levels can trigger qE and CCM genes in the absence of light. WT,cia5andcia5-Ccells were bubbled with air overnight in darkness; next day air bubbling was either maintained or replaced by CO2-limited-air bubbling in the darkness or in the presence of 600 µmol photons m−2s−1light. Sampling was performed after 1 h (RNA) or 4 h (protein).amRNA accumulation ofLHCSR3.1(qE gene) andCAH4, LCIA, LCI1(CCM genes) in WT,cia5andcia5-C. Data were normalized to WT air dark; (n= 3 biological samples, mean ± s.d.). The p-values for the comparisons of WT withcia5andcia5withcia5-Care based on ANOVA Dunnett’s multiple comparisons test of log10 transformed mRNA data as indicated in the graphs (*P< 0.005, **P< 0.01, ***P< 0.001, ****P< 0.0001, ns, not significant). Exact p-values can be found at the Source Data file.bImmunoblot analyses of LHCSR3 and ATPB (loading control) under the indicated conditions. Representative dataset of experiment repeated three times.cImmunoblot analyses of LHCSR3 and ATPB (loading control) of WT samples presented inb. Above the immunoblot shown are the amount of protein loaded per lane and the quantification of LHCSR3 protein accumulation (calculated as LHCSR3 /ATPB ratio) normalized to the air dark conditions. Representative dataset of experiment repeated three times. 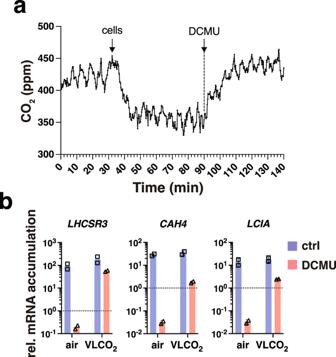Fig. 6: Photosynthetic electron transfer draws down the intracellular CO2concentration, relieving inhibition ofLHCSR3transcription. aCO2concentration measured in the air stream coming out of the headspace of a column filled with 50 mL of HSM, sparged with air under HL. The two arrows in the graph indicate the addition of cells or DCMU.bWT cells were acclimated to LL HSM overnight shaken in flasks; the next day they were exposed to 300 µmol photons m−2s−1light in the presence or absence of 40 µM DCMU, shaken in flasks without or with sparging with VLCO2. Samples were taken after 1 h. Presented are mRNA accumulation ofLHCSR3,CAH4,LCIA. Data were normalized to LL (shown as dotted line in graph);n= 2 biological samples. 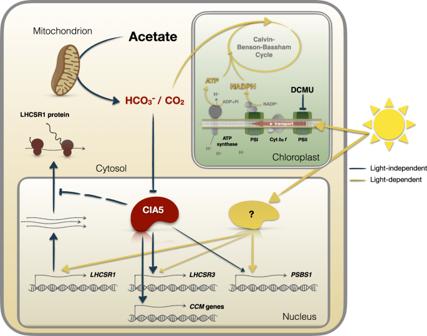Fig. 7: CO2- and light-dependent signals converge to regulate photoprotection and CCM in Chlamydomonas. The intracellular levels of CO2, defined by the equilibrium between CO2fixation in chloroplasts and the generation of CO2by mitochondrial metabolism (e.g. acetate assimilation) is the key determinant of the regulation of gene expression controlling two major processes of photosynthetic organisms: CCM and photoprotection. Changes in light availability have a direct impact on intracellular CO2levels; exposure to HL increases CO2fixation rates leading to depletion of CO2and to activation of not only photoprotection- but also CCM-related genes. Conversely, depletion of CO2is sufficient to drive high expression levels of CCM genes andLHCSR3even in complete darkness (indicated by the black arrows). High CO2levels, either exogenously supplied by sparging or metabolically produced via acetate metabolism or by inhibiting photosynthetic electron flow using DCMU, repressLHCSR3and CCM genes while at the same time they stabilize LHCSR1 protein levels. The close interconnection of photoprotection and CCM is further corroborated by the fact that CIA5, the regulator of expression of genes associated with the CCM, also exerts control overLHCSR3and to a lesser extent overPSBSmRNA levels and acts as repressor of LHCSR1 protein accumulation. Independent of CIA5, light strongly impacts expression of all of these photoprotective genes (yellow arrows). This impact can be the consequence of both photoperception (e.g. phototropin) and the production of reactive oxygen species. Reporting summary Further information on research design is available in the Nature Portfolio Reporting Summary linked to this article.